A facile soft-template synthesis of mesoporous polymeric and carbonaceous nanospheres Owing to the weak self-assembly ability of precursor components and the serious crosslinking of neighbouring nanospheres during a hydrothermal process, the synthesis of monodisperse mesoporous polymer nanospheres with diameters below 500 nm remains a great challenge. Here we extend the synthesis method of mesoporous silica nanospheres to enable the preparation of ordered mesoporous resorcinol formaldehyde nanospheres with particle size from 80 to 400 nm and mesopores of ~3.5 nm in diameter. By finely tuning the synthesis parameters, multi-layered mesoporous resorcinol formaldehyde hollow nanospheres can be successfully synthesized. Mesoporous carbon nanospheres and hollow nanospheres with high surface area are further obtained through carbonization of the polymer spheres. The resulting mesoporous carbon nanospheres are demonstrated as the host cathode material for lithium–sulphur batteries. The synthesis strategy provides a benchmark for fabricating well-defined porous carbonaceous nanospheres with potential for energy storage and conversion applications. The interest in the design and controlled fabrication of nanoporous organic polymers and carbon materials emanates from their tremendous applications in adsorption, catalysis, drug delivery and energy storage/conversion [1] , [2] , [3] , [4] , [5] , [6] , [7] . In particular, polymers and carbon nanoparticles with ordered mesostructures and controlled morphologies have great advantages due to their remarkable and complementary property of the mesochannels and quantum effects in the nanoscale. Many efforts have been made to fabricate mesoporous carbon nanospheres (MCNs) to control their particle size and mesostructures [8] , [9] , [10] , [11] , [12] , [13] , [14] . MCNs can be prepared either through a hard-template method by filling the mesopores of silica template with an organic precursor, or by an organic–organic assembly soft-template method. For example, MCNs with particle sizes of 100–200 nm were successfully synthesized by using a MCM-48-type mesoporous silica nanoparticle as a hard template [8] . Nevertheless, the complicated, high cost, and time-consuming multistep procedure of the hard-template method is a major drawback for its extensive use. In addition, the mesostructures and morphologies of the replicated MCNs are limited to their parent templates [3] , [8] . In contrast, the soft-template method requires fewer synthetic steps than the hard-template method and has proven to be an efficient method for the synthesis of mesoporous phenolic formaldehyde resins polymers and carbons with well-defined pore structures ( Ia3d, p6mm, Im3m, Fd3m and Fm3m ), narrow pore-size distributions and macroscopic morphologies (film, monolith, fibre, sphere and single crystal) [4] , [6] , [7] . However, the particle sizes of the mesoporous carbon spheres fabricated by the aforementioned synthesis methods are large (>1 μm) and not well defined. Until now, only few examples have been reported so far to synthesize MCNs by using the soft-template method, and most of them are unsuitable for large-scale synthesis [12] , [13] , [14] . Zhao and co-workers developed a low-concentration hydrothermal route to synthesize highly ordered body-centered cubic ( Im3m ) MCNs with an uniform particle size (20–140 nm) for the first time [14] , initiating the controlling synthesis of MCNs using the soft-template method. However, this method was a multi-step procedure and needed a large volume of water to dilute the precursor solution, which limited their large-scale synthesis. Therefore, an efficient, facile, general and environmentally friendly method for the synthesis of mesoporous polymer nanospheres (MPNs) and MCNs with ordered mesopores, controllable particle size and morphologies is highly desirable. Recently, we have successfully synthesized polymer spheres by an extended well-known Stöber method; microporous carbon spheres were then obtained by carbonization of the polymer spheres [5] . It suggested that by extending the synthesis method of silica, various nanostructured carbons with different morphologies could be designed and synthesized. Herein we report the synthesis of MCNs by extending the synthesis method of mesoporous silica nanoparticles (Institute of Bioengineering and Nanotechnology, IBN series) [15] . The generation process of MCNs is illustrated in Fig. 1 . The cationic fluorocarbon surfactant FC4, (C 3 F 7 O(CFCF 3 CF 2 O) 2 CFCF 3 CONH(CH 2 ) 3 N + (C 2 H 5 ) 2 CH 3 I − ), and triblock co-polymer Pluronic F127, EO 106 PO 70 EO 106 (EO, ethylene oxide; PO, propylene oxide), are used as templates; ethanol and 1,3,5-trimethylbenzene (TMB) are involved as organic co-solvents; resorcinol and formaldehyde (RF) are selected as carbon precursors. As-synthesized mesoporous RF resins spheres are formed via the assembly of RF together with the emulsion droplets through hydrogen bonding ( Fig. 1 ). MPNs and MCNs are obtained by calcination at 400 °C and 800 °C under N 2 , respectively. The resulted MCNs are investigated as a cathode material and a sulphur host in Li–S batteries which shows high initial discharge capacity and good cyclability. The approach is considered to be efficient, facile, low cost and environmentally friendly for the synthesis of mesoporous polymer and carbon nanopsheres with ordered mesostructure in a high yield, and to be more suitable for industrial production. 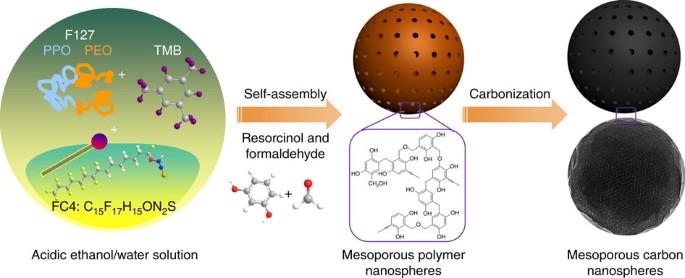Figure 1: Schematic illustration of the formation of MCNs. Self-assembly of mesoporous polymer spheres, followed by carbonization for the synthesis of MCNs. Figure 1: Schematic illustration of the formation of MCNs. Self-assembly of mesoporous polymer spheres, followed by carbonization for the synthesis of MCNs. Full size image Fabrication of MPNs MPNs were synthesized under the similar conditions to the preparation of IBN-1. Without the addition of ethanol, uniform MPNs with disordered mesostructure and particle size around 80 nm was formed ( Supplementary Fig. S1 ). The particle size is smaller than IBN (100–300 nm), and the mesostructure is different from the cubic mesostructure of IBN-1. In order to get ordered mesosturcture, ethanol was added in the synthesis system because ethanol can promote a slow polymerization of RF precursors, which is favourable for the formation of well-defined mesophases by the supra-molecular assembly ( Supplementary Table S1 ). Before the hydrothermal treatment, the reaction solutions changed from pink to yellow colour with increasing the addition amount of ethanol while keeping the other reaction conditions the same, which was related to the oxidation extent of phenolic resins ( Supplementary Fig. S2 ). With increasing the ethanol addition amount (2~19 ml), the particle sizes of the resulted MPNs increased gradually from 80 to 400 nm accompanied with the particles turning to non-uniform ( Supplementary Fig. S1 ). When the ethanol amount reached to 20~26 ml, uniform MPNs with particle size around 400 nm were obtained. Scanning electron microscopy (SEM) images ( Fig. 2a ) show that MPNs-1 synthesized with 26 ml of ethanol are spherical in morphology and has an average particle size of 400 nm. High-resolution SEM (HRSEM) images of MPNs-1 display meat-ball-like morphology with mesopores on the rough surface ( Fig. 2a inset). The corresponding transmission electron microscopy (TEM) images further confirm the spherical morphology and highly ordered mesostructures ( Fig. 2b–d ). The mesostructures of MPNs-1 were further verified by using small-angle X-ray scattering (SAXS) and nitrogen sorption characterization. The SAXS pattern of MPNs-1 shows two well-resolved peaks, which can be indexed as the 10, and 11 reflections of 2D hexagonal ( p6mm ) symmetry with a lattice constant of a =14 nm ( Fig. 2e ). The nitrogen sorption of MPNs-1 shows a typical type-IV isotherm, indicating the presence of uniform channel-like mesopores with a diameter of 3.5 nm ( Fig. 2f,g ). MPNs-1 has a high Brunauer–Emmett–Teller (BET) surface area of 462 m 2 g –1 and a high pore volume of 0.29 cm 3 g –1 . Mesoporous aminophenol formaldehyde nanospheres with average particle size of ~400 nm were further synthesized under the similar preparation conditions to the preparation of MPNs-1 except using aminophenol and formaldehyde as precursors ( Supplementary Fig. S3 ). It is found that the developed synthesis method is general and can be extended to prepare various functional polymeric nanospheres. 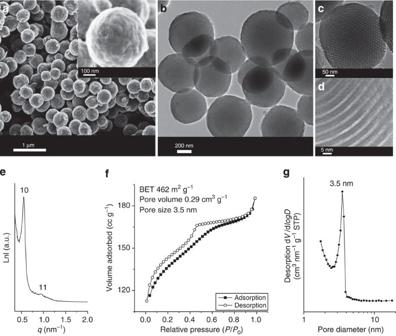Figure 2: Characterization of the mesoporous polymer nanospheres. (a) SEM image, scale bar, 1 μm (inset is HRSEM image, scale bar=100 nm); (b,c) TEM images; (b) scale bar, 200 nm, (c) scale bar, 50 nm; (d) HRTEM image, scale bar, 5 nm; (e) SAXS pattern; (f) nitrogen adsorption desorption isotherms, and (g) pore-size distribution of mesoporous polymer nanospheres (MPNs-1). Figure 2: Characterization of the mesoporous polymer nanospheres. ( a ) SEM image, scale bar, 1 μm (inset is HRSEM image, scale bar=100 nm); ( b , c ) TEM images; ( b ) scale bar, 200 nm, ( c ) scale bar, 50 nm; ( d ) HRTEM image, scale bar, 5 nm; ( e ) SAXS pattern; ( f ) nitrogen adsorption desorption isotherms, and ( g ) pore-size distribution of mesoporous polymer nanospheres (MPNs-1). Full size image Fabrication of multi-shelled hollow MPNs Further increasing the amount of ethanol (27~30 ml), mesoporous polymer hollow nanospheres were generated ( Supplementary Figs S1 and S2 ). MPNs-2 was synthesized under similar preparation conditions to those for MPNs-1, except that more ethanol was added (29 ml) (see Supplementary Table S1 ). SEM images show that MPNs-2 are well-dispersed spherical particles with an average particle size around 350 nm ( Fig. 3a ). HRSEM image of MPNs-2 displays the particles with concave surface ( Fig. 3a inset). TEM images indicate that MPNs-2 has vesicle-like multilayered structures with ordered mesopores ( Fig. 3b–d ). The pore size is estimated to be 3.5 nm by the HRTEM image ( Fig. 3d ). Similar to MPNs-1, MPNs-2 has two well-resolved 10 and 11 reflection peaks in the SAXS pattern which are attributed to 2D hexagonal mesostructures ( Fig. 3e ). The nitrogen sorption of MPNs-2 also shows a typical type-IV isotherm, indicating the presence of uniform channel-like mesopores with a diameter of 3.5 nm ( Fig. 3f,g ). Those results suggest that ethanol has an import role in the formation of vesicles. 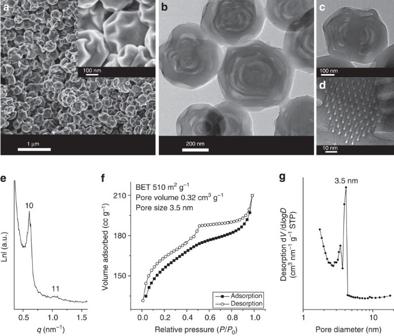Figure 3: Characterization of the multi-shelled hollow mesoporous polymer nanospheres. (a) SEM image; scale bar, 1 μm (inset is HRSEM image; scale bar, 100 nm); (b,c) TEM images; (b) scale bar, 200 nm, (c) scale bar, 100 nm; (d) HRTEM image; scale bar, 10 nm; (e) SAXS pattern; (f) nitrogen adsorption desorption isotherms, and (g) pore-size distribution of multi-shelled hollow mesoporous polymer nanospheres (MPNs-2) which was synthesized with addition of 29 ml ethanol. Figure 3: Characterization of the multi-shelled hollow mesoporous polymer nanospheres. ( a ) SEM image; scale bar, 1 μm (inset is HRSEM image; scale bar, 100 nm); ( b , c ) TEM images; ( b ) scale bar, 200 nm, ( c ) scale bar, 100 nm; ( d ) HRTEM image; scale bar, 10 nm; ( e ) SAXS pattern; ( f ) nitrogen adsorption desorption isotherms, and ( g ) pore-size distribution of multi-shelled hollow mesoporous polymer nanospheres (MPNs-2) which was synthesized with addition of 29 ml ethanol. Full size image Fabrication of MCNs RF resins can convert to carbon with a high yield at high temperature in an inert gas. Thermogravimetric (TG) analyses results ( Supplementary Fig. S4 ) indicate that the carbonization of RF resins starts at 400 °C; therefore, two-step carbonization processes were adapted with pyrolysis of MPNs at 400 °C for 6 h, then carbonization at 800 °C for 6 h in nitrogen flow. MCNs with tuneable mesostructures and morphologies can be directly produced by the carbonization of MPNs ( Supplementary Fig. S5 ). SEM and TEM images ( Fig. 4a,b,d,e and Supplementary Fig. S5 ) show that all the carbon spheres preserve a spherical morphology. Pyrolysis results in ~10% shrinkage from polymer to carbon spheres. Compared with the polymer spheres, mesostructures of the resulted carbon spheres are disordered on a certain extent due to the melt of linear novolac during the pyrolysis and carbonization processes. This can probably be further improved by adding a curing agent such as hexamethyltetramine to achieve ordered mesostructure of the carbon spheres. The porosity of the obtained MCNs was analysed by N 2 sorption. N 2 sorption isotherms of MCNs-1 and MCNs-2 exhibit a intermediate type between type I, which is related to micropores, and type IV, which is related to mesopores, indicating that the samples have the hierarchical porous structures ( Fig. 4c,f ). This finding is in good agreement with TEM observation. The small pore size (3 nm) observed in TEM images is produced owing to the co-template of FC4 and another triblock co-polymer and the crosslinking properties of RF precursors, as well as a large shrinkage of the resin polymer frameworks during the pyrolysis at a high temperature [14] . However, pore size of the resulted carbon nanospheres is tuneable by changing the synthesis parameters such as the concentration of ethanol or TMB. Nitrogen sorption results show that the BET surface areas of MCNs-1 and MCNs-2 are 857 and 640 m 2 g −1 , and the total pore volumes are ~0.45 and 0.34 cm 3 g −1 , respectively ( Supplementary Table S2 ). 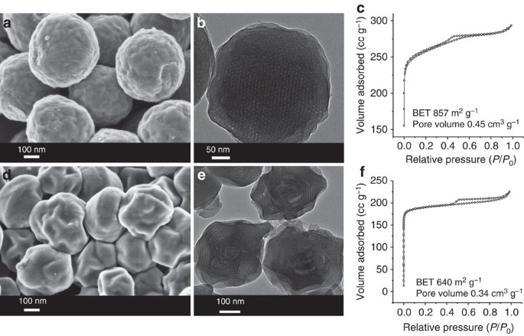Figure 4: Characterization of the MCNs. (a,d) HRSEM images; scale bar, 100 nm, (b,e) TEM images; (b) scale bar, 50 nm, (e) scale bar, 100 nm; (c,f) nitrogen adsorption desorption isotherms ofa,b,cMCNs-1, andd,e,fMCNs-2. Figure 4: Characterization of the MCNs. ( a , d ) HRSEM images; scale bar, 100 nm, ( b , e ) TEM images; ( b ) scale bar, 50 nm, ( e ) scale bar, 100 nm; ( c , f ) nitrogen adsorption desorption isotherms of a , b , c MCNs-1, and d , e , f MCNs-2. Full size image Li–S batteries and electro-catalysis Nanoporous carbon has been recognized as an advanced sulphur immobilizer for Li–S batteries [10] , [16] , [17] , [18] , [19] , [20] , [21] , [22] . The resultant carbon nanospheres with periodically engineered mesostructure were mixed with sulphur following a melt-diffusion strategy to produce MCNs@S which was used as a sulphur cathode in this work. TG measurement in N 2 was carried out to determine S content in the composites ( Supplementary Fig. S6a ). MCNs-1@S composite exhibits the first weight loss from 160 to 360 °C. The sulphur content of MCNs-1@S composite is calculated to be ~20 wt% ( Supplementary Fig. S6a,b ). The morphology and mesostructure have not changed after the sulphur loading based on the observation of TEM images ( Supplementary Fig. S6c,d ). The galvanostatic charge–discharge capacity of MCNs-1@S is shown in Fig. 5a . The discharge capacity recorded at 0.09C in the first cycle is about 1200, mAh g −1 . Note that the initial capacity of sulphur measured below 1.7 V is primarily contributed by the irreversible electrochemical decomposition of LiNO 3 [20] , [23] . Therefore, the capacity of 850 mAh g −1 (red curve in Fig. 5a ) from the second cycle is more meaningful, which preserves ~51% of the theoretical value of sulphur (1672, mAh g −1 ). By a 20 times increment of current density from 0.09 to 1.8 C, the discharge capacity keeps at 400 mAh g −1 ( Fig. 5b ), indicating the high rate performance due to the intimate contact of sulphur with the mesostructured carbon. In a short word, this mesostructured C–S composite promises the use as a cathode in Li–S batteries. 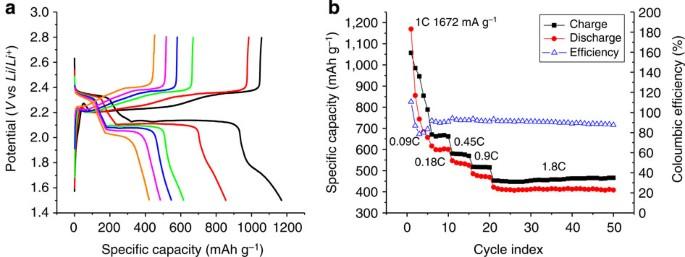Figure 5: Lithium–sulphur battery properties for MCNs as host cathode material. (a) Galvanostatic charge–discharge curves of the S–C composite at different C rates (1C=1672, mA g−1). Black, first cycle at 0.09C; red, second cycle at 0.09C; green, first cycle at 0.18C; blue, first cycle at 0.45C; pink, first cycle at 0.9C; yellow, first cycle at 1.8C; and (b) cycling stability and coloumbic efficiency at different C rates. Figure 5: Lithium–sulphur battery properties for MCNs as host cathode material. ( a ) Galvanostatic charge–discharge curves of the S–C composite at different C rates (1C=1672, mA g −1 ). Black, first cycle at 0.09C; red, second cycle at 0.09C; green, first cycle at 0.18C; blue, first cycle at 0.45C; pink, first cycle at 0.9C; yellow, first cycle at 1.8C; and ( b ) cycling stability and coloumbic efficiency at different C rates. Full size image The resulted MCNs were further tested as metal-free catalysts for oxygen reduction reaction (ORR), which showed good catalytic performance ( Supplementary Fig. S7 ). On the ORR polarization curves, MCNs-1 shows a much better ORR activity than natural graphite powder. Therefore, enhanced ORR activity would be predicted by engineering MCNs-1 through hetero-atom incorporation. In addition, Pt-loaded MCNs-1 ( Supplementary Fig. S8 ) is very active for the hydrogen evolution reaction (HER). Considering the relative low Pt-loading amount (2.3 wt% and 4.6 μg cm −2 of MCNs-1), its catalytic performance for HER is fairly good. All the above application results indicate the obtained MCNs have promising applications in energy storage and conversion. To understand the formation mechanism, the effect of TMB amount, concentration of FC4, and initial synthesis temperatures (ISTs) on the morphology evolution of MPNs was investigated ( Supplementary Table S1 ). The results suggested that higher FC4 or TMB concentrations were favourable for the formation of multilayer hollow structures ( Supplementary Figs S9 and S10 ). RF polymer resins synthesized in the absence of TMB are all composed of solid microspheres with size around 2 μm ( Supplementary Fig. S9 ), implying that TMB acted not only as a swelling agent for F127 micelles but also as a co-solvent for the formation of vesicular structures. The role of TMB was further confirmed by the TEM image results of the samples in the absence of ethanol ( Supplementary Fig. S11 ). MPNs synthesized at higher FC4 concentration showed the vesicular structures. Furthermore, the effect of ISTs on morphology and mesostructures was investigated under the same synthesis condition of MPNs-1. At a lower IST of 20 °C, multi-shelled hollow polymer spheres were obtained. With increasing IST to 50 °C, 100 nm MPNs with ordered mesostructures and larger pore size (14 nm) were produced ( Supplementary Fig. S12 ). The formation of samples with various morphology and mesostructure is probably due to the different FC4 and F127 surfactant phases formed at different temperature. At a low temperature (20 °C), the methyl groups of the PO blocks become hydrated and they form vesicle structures with FC4 and TMB. At a high temperature (50 °C), the interaction between PO group and water is reduced, and TMB can swell the PO chains to make the micelle size increasing. Therefore, MPNs with a larger pore size can be obtained, indicating that the pore sizes of MPNs and MCNs are tuneable by changing the synthesis parameters [15] , [24] , [25] . The transformation from mesoporous nanospheres to multi-layer concave hollow nanospheres, either with increasing amount of ethanol and TMB, concentration of FC4, or decreasing the IST, can be explained by the thermodynamic change of the surfactant hydrophobicity. Generally, the formation of multilamellar vesicles with a desired number of layers depends on the competition between bending energy and layer-to-layer interactions [24] . Hydrophobic PO segments of Pluronic F127 can interact with TMB to stabilize the oil/water emulsion generated in a high ethanol concentration. The vesicles with multilayered structures are formed owing to the decrease of the bending energy. RF precursors interact with vesicles through hydrogen bonds to co-assemble multi-lamellar mesostructure at the oil/water emulsion interface formed by ethanol, TMB, FC4 and F127. It has been reported that multi-shelled hollow silicas can be formed from the vesicles of FC4 and F127 under a similar condition [24] . Ethanol is noted as a good solvent for EO part of F127 but a non-solvent for PO blocks. The morphology transformation can be attributed to the selective swelling of the dispersed EO domains and the slight plastic deformation of non-swelling PO matrix with variation of ethanol concentration. With a low concentration of ethanol, MPNs were formed by the self-assembly of RF and F127 micelles. The spherical vesicle would be formed quickly at a high concentration of ethanol in the presence of TMB, and the inward stress can be generated between the F127 micelle surfaces and the RF frameworks. Meanwhile, water molecules would penetrate outwardly from the cavities of the vesicles under the inward stress, which would cause vesicle deformation, resulting in a concave morphology [24] , [25] . In summary, nanospheres or hollow nanospheres of highly ordered mesoporous polymers and porous carbons with tuneable particle size have been successfully synthesized by the soft-template method. The morphology, pore size and functionality of the resulted mesoporous carbon can all be well adjusted by precise tuning of the synthesis parameters. These carbon materials have a variety of properties, and their application potential for energy storage and conversion has been tested. The polymer and carbon spheres developed in this work are potentially important for various applications such as electrode materials, photonics, separation, water treatment and drug delivery. Synthesis of MPNs and MCNs In a typical synthesis, 1.0 g of Pluronic F127, 0.2 g of FC4 and 1.0 g of KCl were dissolved in 60 ml of 2 M HCl at 30 °C under vigorous stirring, followed by the introduction of 1.0 g of 1,3,5-TMB and desired amount of ethanol (2~40 ml). When the co-polymer was fully dissolved, formaldehyde solution (0.56 ml) and resorcinol (0.4 g) was added to the reaction solution and stirred for 24 h at 30 °C, and subsequently heated for 24 h at 100 °C under a static condition in a Teflon-lined autoclave. The solid product was recovered by centrifugation and air-dried at 100 °C for 48 h. The obtained MPNs were heated at 400 °C for 2 h with a rate of 5 °C min −1 in nitrogen flow to remove the template. MCNs were produced by a direct carbonization of as-made MPNs at 400 °C for 6 h, then at 800 °C for 6 h in nitrogen flow with a heating rate of 1.5 °C min −1 . Synthesis of Pt-deposited MCNs-1 100 mg MPNs-1 was dispersed into 10 ml of 10 mM H 2 PtCl 6 solution, and the resulted solution was stirred overnight in an ultrasonic water bath. The powers were collected by centrifuging, and dried at 100 °C overnight. Pt@MCNs-1 was obtained through pyrolysis of the above powders in tube furnace from 50 to 700 °C in flowing N 2 at a heating rate of 1 °C min −1 . The Pt-loading amount is 2.3 wt% according to the TG results. Characterization X-ray diffraction patterns at low (0.5–5° in 2 θ ) were collected on a D8-ADVANCE powder X-ray diffractometer operation at 40 kV and 30 mA using Cu-K α radiation ( λ =0.15406, nm). Nitrogen-sorption isotherms were collected by Tristar II, Micromeritics nitrogen sorption analyser at 77 K. Prior to the measurement, samples were degassed at 120 °C for at least 10 h. The BET specific surface area was calculated using adsorption data at a relative pressure range of P / P 0 =0.05–0.25. Pore-size distribution was derived from the desorption branch using Barrett–Joyner–Halenda method. The total pore volume was estimated from the adsorbed amounts at a relative pressure ( P / P 0 ) of 0.99. SEM was taken with a Hitachi Model S-4800 field emission electron microscopy operating at 8 kV. TEM measurements were conducted on a JEM-2100 F microscope (JEOL, Japan) operated at 200 kV. The samples for TEM measurement were suspended in ethanol and supported onto a holey carbon film on a Cu grid. The amount of sulphur in the composites was determined by TG analyses using a Perkin-Elmer TGA 7 TG analyser from 25 to 800 °C in flowing N 2 at a heating rate of 10 °C min −1 . Electrochemical measurements The MCNs/S nanocomposite was prepared following a melt-diffusion strategy by grounding together, and heating to 155 °C. Sulphur–carbon composite cathodes were made by 80 wt% MCNs/S nanocomposite, 10 wt% carbon black and 10 wt% poly(vinylidene fluoride) binder. The cathode materials were slurry-cast from N-methyl-2-pyrrolidone onto an aluminium foil current collector. The electrolyte was composed of a 1.0 M lithium bis-trifluoromethanesulfonylimide in 1,3-dioxolane and 1,2-dimethoxyethane (1:1 by volume) with 0.5 wt% LiNO 3 additive. A 2032-type stainless steel coin cell was used to assemble the half-cell for testing. A lithium metal foil was used as an anode, and the sulphur–carbon composite on aluminium foil was a cathode. A LAND galvanostatic charge-discharge cycle instrument was used to perform the measurements. The coin-type cell was assembled in an Ar-filled glove box (MBraun Unilab). ORR measurements ORR activity was determined in 0.1 M KOH solution saturated with oxygen. Cyclic voltammetry was collected in the nitrogen and oxygen saturated solutions, respectively, at a scan rate of 50 mV/s. Rotating disk electrode voltammetry was measured at 10 mV s −1 at a rotating speed from 400 to 1200 r.p.m. Potential range is set from −1.25 to 0.25 V versus Hg/HgO. HER measurements In a typical electrochemical measurement, 2 mg of Pt loaded MCNs-1 powder is dispersed in 1 ml 0.1% Nafion aqueous solution by ultrasonication. Twenty microlitre of the dispersion is dipped on a 5 mm diameter glassy carbon electrode and dried in ambient environment. The catalyst loading on the electrode is about 200 mg cm −2 . The Pt loading is 4.6 μg cm −2 . 0.5 M H 2 SO 4 aqueous solution, a Ag/AgCl electrode (4 M KCl, 0.2 V versus standard hydrogen electrode) and a Pt wire are used as the electrolyte, reference electrode and counter electrode, respectively. The electrolyte is saturated with N 2 of 1 atm. How to cite this article: Liu, J. et al. A facile soft-template synthesis of mesoporous polymeric and carbonaceous nanospheres. Nat. Commun. 4:2798 doi: 10.1038/ncomms3798 (2013).